Reconciliation of marine and terrestrial carbon isotope excursions based on changing atmospheric CO2levels Negative carbon isotope excursions measured in marine and terrestrial substrates indicate large-scale changes in the global carbon cycle, yet terrestrial substrates characteristically record a larger-amplitude carbon isotope excursion than marine substrates for a single event. Here we reconcile this difference by accounting for the fundamental increase in carbon isotope fractionation by land plants in response to increasing atmospheric CO 2 concentration ( p CO 2 ). We show that for any change in p CO 2 concentration (Δ p CO 2 ), terrestrial and marine records can be used together to reconstruct background and maximum p CO 2 levels across the carbon isotope excursion. When applied to the carbon isotope excursion at the Palaeocene–Eocene boundary, we calculate p CO 2 =674–1,034 p.p.m.v. during the Late Palaeocene and 1,384–3,342 p.p.m.v. during the height of the carbon isotope excursion across all sources postulated for the carbon release. This analysis demonstrates the need to account for changing p CO 2 concentration when analysing large-scale changes in the carbon isotope composition of terrestrial substrates. Globally correlated, negative excursions in carbon isotope (δ 13 C) values measured in marine and terrestrial substrates throughout the Phanerozoic indicate episodic, massive additions of isotopically depleted carbon to the ocean–atmosphere system [1] , [2] , [3] , [4] , [5] , [6] , [7] , [8] , [9] , [10] . These events not only changed the carbon isotope composition of atmospheric carbon dioxide (δ 13 C CO2 ), but also raised p CO 2 concentrations (for example, ref. 11 ). The magnitude of the carbon isotope excursion (CIE) and the amount of p CO 2 rise (Δ p CO 2 ) calculated for such events should relate to one another, and the source of the carbon input and changes in the global carbon cycle have been reconstructed upon this premise (for example, refs 5 , 9 , 11 , 12 ). Determination of the ‘true’ magnitude of a CIE (that is, the amount of the CIE caused only by the change in δ 13 C CO2 ) is fundamental to calculating the amount of carbon added to the atmosphere at the event and improving our understanding of feedbacks in the climate system [13] , [14] . One complicating factor is that the magnitude of the CIE is characteristically larger when measured in terrestrial versus marine substrates by up to several per mil [6] , [7] , [8] , [9] , [11] , [15] . Workers have argued that larger-magnitude negative excursions recorded in terrestrial substrates reflect increased humidity or precipitation [6] , [7] based on the increased carbon isotope fractionation that modern land plants demonstrate in response to these environmental factors. Others have attributed this difference to an increased abundance of angiosperm flora, which are characteristically isotopically depleted in comparison with gymnosperm flora [16] , [17] . Both of these mechanisms are problematic as general explanations for any global discrepancy between terrestrial and marine CIEs because their influences are most likely to be locally and heterogeneously expressed [15] , [18] ( Supplementary Information ). Moreover, changes in angiosperm abundance cannot explain larger terrestrial versus marine CIEs in pre-Cretaceous substrates (for example, ref. 7 ). The reconciliation of terrestrial versus marine CIEs requires a mechanism fundamental to all C 3 photosynthesis, and thus globally applicable (we note that classical C 4 photosynthesis is a recent evolutionary innovation, relegated to no more than the last ~13 million years of Earth’s history [19] , [20] , and that CAM photosynthesis is largely limited to aqueous and desert environments). Previous experiments have shown that the carbon isotope value of plant tissues (δ 13 C p ) is affected by changes in p CO 2 concentration, independent of changes in δ 13 C CO2 , and identified a positive relationship between p CO 2 concentration and carbon isotope fractionation (Δδ 13 C p ≈δ 13 C CO2 −δ 13 C p ) in both angiosperm and gymnosperm taxa (for example, refs 21 , 22 ; Supplementary Information ). More recently, time-series correlations between climate variables and tree-ring Δδ 13 C p values have been shown to improve when a correction proportional to the increase in p CO 2 is applied (for example, refs 23 , 24 , 25 ). However, a wide range of corrections for the effect of changing p CO 2 on Δδ 13 C p ( S ; ‰/p.p.m.v.) have been reported and applied, typically ranging from S =0.73 to 2.0‰ per 100 p.p.m.v. increase in p CO 2 (for example, refs 23 , 24 ; Supplementary Information ). Our recent work growing plants under controlled environmental conditions across a wide range of p CO 2 levels (up to 4,200 p.p.m.v.) provided a unifying relationship for the effect of p CO 2 on C 3 plant tissue, showing that S decreases systematically with increasing p CO 2 across a wide range of C 3 plants ( R =0.96, n =33) ( Fig. 1 ) ( [26] ). This relationship suggests that for any large release of isotopically depleted carbon to the ocean or atmosphere, the land-plant-derived substrates of the terrestrial record (CIE terrestrial ; that is, terrestrial organic matter, soil carbonate, plant lipids and tooth enamel) will record a larger-amplitude CIE than marine substrates (CIE marine ; that is, benthic foraminifera, planktic foraminifera and bulk marine carbonate). Thus, we propose that the difference in magnitude between these two substrates (ΔCIE=CIE terrestrial −CIE marine ) results from the additional fractionation by land plants due to rising p CO 2 levels, which is then propagated within the terrestrial record. We apply this to the particularly well-studied and globally widespread CIE at the Palaeocene–Eocene Thermal Maximum (PETM), for which analysis of >150 CIEs shows a significant, 2.1‰ greater amplitude CIE recorded in terrestrial versus marine substrates [11] , in order to calculate absolute p CO 2 levels during the Late Palaeocene and at the height of the CIE for the range of sources (and thus, Δ p CO 2 values) postulated for the carbon release. 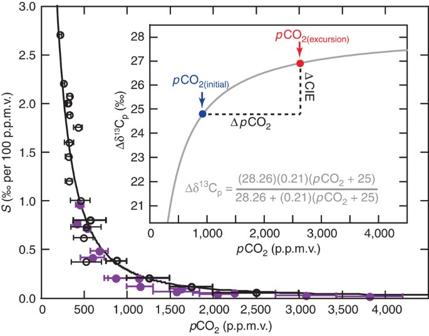Figure 1: The effect ofpCO2concentration on C3land-plant carbon isotope fractionation. Across field and chamber experiments on a wide range of C3land-plant species, the amount of carbon-isotope fractionation per change inpCO2(S, ‰ per p.p.m.v.) decreases within increasingpCO2level according to the following equation:S=(B)(A2)/[A+B(pCO2+C)]2withR=0.96 (n=33) (black curve), whereA=28.26,B=0.21 andC=25. Purple closed circles reflect data from our experiments26; open black circles represent data compiled from published studies (Supplementary Table S2). Horizontal bars encompass the range ofpCO2levels used within each experiment; the circle is plotted at the midpoint of the range. The grey curve (inset) represents the integral of the black curve, and follows the general hyperbolic relationship: Δδ13Cp=[(A)(B)(pCO2+C)]/[A+(B)(pCO2+C)] (seeSupplementary Information). As the relationship betweenpCO2and Δδ13Cpis nonlinear, absolute estimates ofpCO2(initial)(blue) andpCO2(excursion)(red) can be calculated by solving equations (1) and (2) provided ΔpCO2and ΔCIE are known (dashed lines); for a given magnitude CIE, the ΔpCO2estimate is dependent on the δ13C value of the source. Figure is modified from26with new data reported in Lomaxet al.59(Supplementary Information;Supplementary Table S1). Figure 1: The effect of p CO 2 concentration on C 3 land-plant carbon isotope fractionation. Across field and chamber experiments on a wide range of C 3 land-plant species, the amount of carbon-isotope fractionation per change in p CO 2 ( S , ‰ per p.p.m.v.) decreases within increasing p CO 2 level according to the following equation: S =( B )( A 2 )/[ A + B ( p CO 2 + C )] 2 with R =0.96 ( n =33) (black curve), where A =28.26, B =0.21 and C =25. Purple closed circles reflect data from our experiments [26] ; open black circles represent data compiled from published studies ( Supplementary Table S2 ). Horizontal bars encompass the range of p CO 2 levels used within each experiment; the circle is plotted at the midpoint of the range. The grey curve (inset) represents the integral of the black curve, and follows the general hyperbolic relationship: Δδ 13 C p =[( A )( B )( p CO 2 + C )]/[ A +( B )( p CO 2 + C )] (see Supplementary Information ). As the relationship between p CO 2 and Δδ 13 C p is nonlinear, absolute estimates of p CO 2(initial) (blue) and p CO 2(excursion) (red) can be calculated by solving equations (1) and (2) provided Δ p CO 2 and ΔCIE are known (dashed lines); for a given magnitude CIE, the Δ p CO 2 estimate is dependent on the δ 13 C value of the source. Figure is modified from [26] with new data reported in Lomax et al. [59] ( Supplementary Information ; Supplementary Table S1 ). Full size image Reconciliation of ΔCIE via the p CO 2 effect The larger-magnitude CIE recorded in terrestrial versus marine substrates can be described by the following equation relating ΔCIE to the effect of changing p CO 2 levels on carbon isotope fractionation by C 3 land plants: where p CO 2(initial) and p CO 2(excursion) are the p CO 2 levels immediately before and at the height of the CIE, respectively, and A , B and C are constants produced by the best-fit curve through the experimental data and published values ( Fig. 1 inset and Supplementary Information ). For CIE events where the magnitude of both CIE terrestrial and CIE marine are well-documented globally, knowledge of ΔCIE can be used towards the determination of both p CO 2(initial) and p CO 2(excursion) provided the change in p CO 2 (Δ p CO 2 ) is known ( Fig. 1 inset): Estimates of Δ p CO 2 , which are dependent on the true magnitude of the CIE and the δ 13 C value of the source (δ 13 C source ), are commonly calculated using methods ranging from mass balance equations (for example, refs 5 , 11 ) to numerical models (for example, refs 12 , 27 ). Therefore, provided independent estimates of ΔCIE and Δ p CO 2 , equations (1) and (2) can be solved simultaneously for absolute estimates of p CO 2(initial) and p CO 2(excursion) ( Fig. 2 ), allowing for a wholly new quantitative reconstruction of changes in the global carbon cycle. Although determination of p CO 2(initial) and p CO 2(excursion) requires precise estimates of ΔCIE and Δ p CO 2 , Fig. 2 shows that the value for p CO 2(initial) is more sensitive to ΔCIE than to Δ p CO 2 , while p CO 2(excursion) is more sensitive to Δ p CO 2 than to ΔCIE. 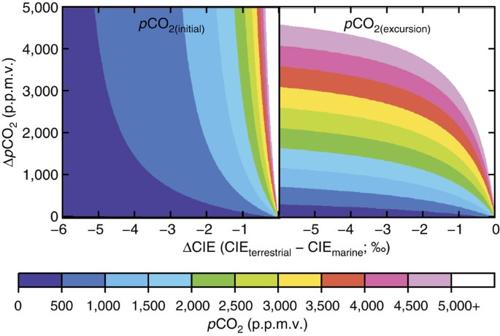Figure 2: Determination ofpCO2levels as a function of ΔCIE and ΔpCO2. For any hypothetical CIE,pCO2(initial)(left) andpCO2(excursion)(right) are a function of the difference between the terrestrial and marine CIE (ΔCIE; ΔCIE=CIEterrestrial−CIEmarine) and the rise inpCO2(ΔpCO2; ΔpCO2=pCO2(excursion)−pCO2(initial)). Values forpCO2(initial)andpCO2(excursion)were calculated by solving equations (1) and (2) simultaneously. Figure 2: Determination of p CO 2 levels as a function of ΔCIE and Δ p CO 2 . For any hypothetical CIE, p CO 2(initial) (left) and p CO 2(excursion) (right) are a function of the difference between the terrestrial and marine CIE (ΔCIE; ΔCIE=CIE terrestrial −CIE marine ) and the rise in p CO 2 (Δ p CO 2 ; Δ p CO 2 = p CO 2(excursion) − p CO 2(initial) ). Values for p CO 2(initial) and p CO 2(excursion) were calculated by solving equations (1) and (2) simultaneously. Full size image Determination of p CO 2 levels across the CIE at the PETM The highly studied, globally widespread CIE that marks the PETM represents an ideal event upon which to first apply our methods to quantify p CO 2(initial) and p CO 2(excursion) because of the large number of CIE terrestrial and CIE marine records that can be used to provide a robust estimate of ΔCIE globally. More than 150 total CIE marine and CIE terrestrial records have been measured across the PETM (reviewed by McInerney and Wing [11] ); the average CIE measured in terrestrial substrates that include soil carbonate, plant lipids, bulk soil organic matter and tooth enamel (CIE terrestrial ±1 σ =−4.7±1.5‰, n =48) is 2.1‰ more negative than that measured in benthic foraminifera, planktic foraminifera and bulk marine carbonate from marine environments (CIE marine ±1 σ =−2.6±1.1‰, n =105) (ΔCIE=−2.1‰). Bulk marine organic matter was not included in our determination of CIE marine because it can include mixed pools of carbon from photosynthetic and non-photosynthetic organisms from terrestrial and marine environments [15] , [28] , [29] , [30] . By averaging across the large number of diverse sites and substrates available for the PETM, biasing effects of local and regional changes in climate [6] , [8] , [31] , [32] , [33] , [34] , [35] , [36] , [37] , [38] , [39] , vegetation [16] , [17] , [38] , sediment transport [40] , [41] , salinity [15] , [42] and dissolution [43] , [44] on ΔCIE are limited. Using this ΔCIE value (−2.1‰), Late Palaeocene ( p CO 2(initial) ) and PETM ( p CO 2(excursion) ) p CO 2 levels can be determined across a range of Δ p CO 2 estimates by simultaneously solving equations (1) and (2) ( Fig. 3 ). 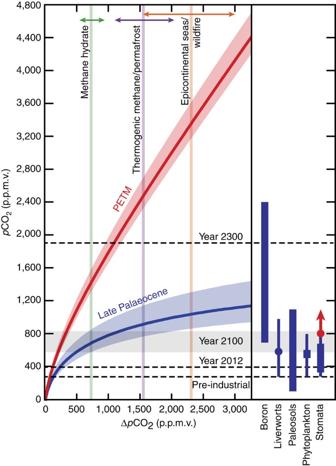Figure 3: Reconstruction ofpCO2levels during the Late Palaeocene and PETM. Across a range of possiblepCO2increases (ΔpCO2),pCO2levels for the Late Palaeocene (blue curve;pCO2(initial)) and PETM (red curve;pCO2(excursion)) were calculated by simultaneously solving equations (1) and (2) for ΔpCO2=0–3,600 p.p.m.v. and ΔCIE=−2.1‰ (thick curves). Blue and red shaded regions show solutions for ΔCIE=−1.6 to −2.6‰ to illustrate the effect of ΔCIE onpCO2estimates (for a given ΔpCO2, lower ΔCIE values yield higherpCO2estimates andvice versa). ΔCIE=−2.5‰ assumes thatn-alkanes (CIE=−5.1‰;11) best represent CIEterrestrial; ΔCIE=−1.6‰ suggests a smaller offset between CIEterrestrialand CIEmarineowing to an underestimation of the magnitude of CIEmarine(CIEmarine=−3.1‰ versus −2.6‰). Vertical lines mark ΔpCO2estimates for specific proposed sources of the event (green=methane hydrate14, δ13Csource=−60‰; purple=thermogenic methane54or permafrost thawing50, δ13Csource=−30‰; and orange=wildfire burning55or oxidation of organic matter from drying of epicontinental seas56, δ13Csource=−22‰) based on a mass balance equation (equation (3) and the parameters used by McInerney and Wing11(0.3 p.p.m.v. increase inpCO2per Pg C added, δ13Cinitial=−2.5‰, andMinitial=50,000 Pg C); horizontal arrows mark the range of ΔpCO2estimates calculated for each source (equation (3)), provided a range of estimates for thepCO2increase per Pg C added (0.23 to 0.39) and estimates of δ13Cinitial(−2.5 to −0.1‰) (Methods). The range of average Late Palaeocene (60–55Ma)pCO2estimates from other proxies (blue bars) are indicated; a singlepCO2estimate from stomata provides a lower bound onpCO2during the PETM (red point and arrow) (references are provided in theSupplementary Information). Dashed lines mark pre-industrial (280 p.p.m.v.) and present-day (393 p.p.m.v.)pCO2levels, as well as a model-based projection ofpCO2in the year 2300 if fossil fuel burning continues unabated (1,900 p.p.m.v.) (46). Grey-shaded region represents the range ofpCO2projections for the year 2100 from the IPCC (566–821 p.p.m.v.) (60). Figure 3: Reconstruction of p CO 2 levels during the Late Palaeocene and PETM. Across a range of possible p CO 2 increases (Δ p CO 2 ), p CO 2 levels for the Late Palaeocene (blue curve; p CO 2(initial) ) and PETM (red curve; p CO 2(excursion) ) were calculated by simultaneously solving equations (1) and (2) for Δ p CO 2 =0–3,600 p.p.m.v. and ΔCIE=−2.1‰ (thick curves). Blue and red shaded regions show solutions for ΔCIE=−1.6 to −2.6‰ to illustrate the effect of ΔCIE on p CO 2 estimates (for a given Δ p CO 2 , lower ΔCIE values yield higher p CO 2 estimates and vice versa ). ΔCIE=−2.5‰ assumes that n -alkanes (CIE=−5.1‰; [11] ) best represent CIE terrestrial ; ΔCIE=−1.6‰ suggests a smaller offset between CIE terrestrial and CIE marine owing to an underestimation of the magnitude of CIE marine (CIE marine =−3.1‰ versus −2.6‰). Vertical lines mark Δ p CO 2 estimates for specific proposed sources of the event (green=methane hydrate [14] , δ 13 C source =−60‰; purple=thermogenic methane [54] or permafrost thawing [50] , δ 13 C source =−30‰; and orange=wildfire burning [55] or oxidation of organic matter from drying of epicontinental seas [56] , δ 13 C source =−22‰) based on a mass balance equation (equation (3) and the parameters used by McInerney and Wing [11] (0.3 p.p.m.v. increase in p CO 2 per Pg C added, δ 13 C initial =−2.5‰, and M initial =50,000 Pg C); horizontal arrows mark the range of Δ p CO 2 estimates calculated for each source (equation (3)), provided a range of estimates for the p CO 2 increase per Pg C added (0.23 to 0.39) and estimates of δ 13 C initial (−2.5 to −0.1‰) (Methods). The range of average Late Palaeocene (60–55Ma) p CO 2 estimates from other proxies (blue bars) are indicated; a single p CO 2 estimate from stomata provides a lower bound on p CO 2 during the PETM (red point and arrow) (references are provided in the Supplementary Information ). Dashed lines mark pre-industrial (280 p.p.m.v.) and present-day (393 p.p.m.v.) p CO 2 levels, as well as a model-based projection of p CO 2 in the year 2300 if fossil fuel burning continues unabated (1,900 p.p.m.v.) ( [46] ). Grey-shaded region represents the range of p CO 2 projections for the year 2100 from the IPCC (566–821 p.p.m.v.) ( [60] ). Full size image Reconstructed estimates of p CO 2(initial) and p CO 2(excursion) increase as Δ p CO 2 increases ( Fig. 3 ); thus the solution based on a methane hydrate source (δ 13 C source =−60‰, Δ p CO 2 =710 p.p.m.v.) yielded the lowest Late Palaeocene p CO 2 estimate ( p CO 2(initial) =674 p.p.m.v. ), followed by thermogenic methane or permafrost thawing (δ 13 C source =−30‰, Δ p CO 2 =1,566 p.p.m.v.) that yielded p CO 2(initial) =915 p.p.m.v., and then wildfire or drying of epicontinental seas (δ 13 C source =−22‰, Δ p CO 2 =2,308 p.p.m.v.) having the highest Late Palaeocene p CO 2 estimate ( p CO 2(initial) =1,034 p.p.m.v.). If these sources can be thought to exhaust the carbon isotope range of potential sources, we calculate that Late Palaeocene p CO 2 levels may have been as low as ~280 p.p.m.v. higher than present, and were much lower than the recent p CO 2 estimates for the year 2300 ( [45] , [46] ; Fig. 3 ). p CO 2 levels at the peak of the PETM were calculated to be 1,384, 2,481 and 3,342 p.p.m.v. for methane hydrate, thermogenic methane or permafrost thawing, and drying of epicontinental seas or wildfire sources (Δ p CO 2 =710, 1,566 and 2,308 p.p.m.v. ), respectively ( Fig. 3 ). Determination of Late Palaeocene and PETM p CO 2 levels is important for quantifying climate sensitivity to CO 2 for this greenhouse period (for example, ref. 47 ); however, previous proxy estimates for the Late Palaeocene are highly varied, ranging from 100 to 2,400 p.p.m.v., and robust PETM p CO 2 estimates are lacking ( Supplementary Information ; Fig. 3 ). Across a wide range of increases in p CO 2 at the PETM (Δ p CO 2 ≤ 3,000 p.p.m.v. ), our results indicate that Late Palaeocene p CO 2 levels were≤1,112 p.p.m.v. ( Fig. 3 ). If we consider a relatively small increase in p CO 2 levels (Δ p CO 2 <1,000 p.p.m.v. ), as would be attributed to a methane hydrate source, our Late Palaeocene p CO 2 estimates are consistent with values determined from liverwort, phytoplankton and stomatal proxies ( Fig. 3 ). The boron isotope proxy, in contrast, is more consistent with our results assuming that the amount of p CO 2 increase was larger (>1,000 p.p.m.v. ), as would be required for the thawing permafrost model, for example ( Fig. 3 ). Although our reconciliation does not allow for the determination of the carbon source of the CIE at the PETM, recent work indicates significant warming before the onset of the CIE ( [33] , [48] ), and suggests an orbitally forced mechanism for the release of carbon at the event [49] , [50] , [51] . If we consider the two hypotheses suggesting that orbital forcing triggered the release of carbon through a methane hydrate release ( [49] ) (Δ p CO 2 =710 p.p.m.v.) or large-scale thawing of permafrost ( [50] ) (Δ p CO 2 =1,566 p.p.m.v. ), we calculate Late Palaeocene p CO 2 levels=674 (+159−109) or 915 (+225−153) p.p.m.v., respectively (error based on ΔCIE=−1.6 to −2.6‰; Fig. 3 ). Notably, these calculated values for Late Palaeocene p CO 2 are consistent with the p CO 2 levels required by Lunt et al . [49] (~560 p.p.m.v.) and DeConto et al. [50] (~900 p.p.m.v.) for each of their respective models. Many arguments have been made to explain the larger CIE measured in terrestrial versus marine substrates at the PETM [6] , [8] , [15] , [16] , [17] , [18] , [42] , [43] , but each requires additional phenomena secondary to the carbon release ( Supplementary Information ). Based on the fundamental observation of increased carbon isotope fractionation in C 3 land plants in response to elevated p CO 2 levels ( Fig. 1 ), we propose that the larger amplitude CIE recorded in terrestrial substrates results from the primary phenomenon of rising p CO 2 levels. We attribute deviations from the average size of the CIE measured on the same substrate at different sites to local or regional changes in water availability [6] , [8] , [18] , [36] , plant composition [16] , [17] , [38] , [52] , dissolution [43] and salinity [42] . For these reasons, the average of many CIEs measured across the planet should be used to determine the average magnitude of the marine and terrestrial signals for the purpose of reconciling the magnitude of the event and reconstructing p CO 2 levels. We further note systematic differences in the magnitude of the CIE within the marine and terrestrial substrates as compiled by McInerney and Wing [11] in their Table 1. Within the marine record, foraminifera (benthic and planktonic) and bulk marine carbonate record the smallest CIE (−2.5 to −2.7‰), while algal lipids and bulk marine organic matter record a greater CIE (−3.5 to −4.1‰). In terrestrial systems, the smallest CIE is measured in bulk soil organic matter (−3.5‰), followed by tooth enamel and plant lipids (−4.8 to −5.1‰), with the largest CIE measured in soil carbonate (−5.5‰). The greater CIE measured in algal lipids compared with foraminifera is likely caused by elevated p CO 2 levels, as photosynthetic algae are also known to show increasing carbon isotope fractionation with increasing concentrations of CO 2 dissolved in water although these relationships vary widely (reviewed within ref. 53 ) and differ from that of higher land plants. Bulk organic matter in terrestrial and marine environments show the same median magnitude CIE (−3.5‰); the CIE measured in terrestrial bulk organic matter may be dampened relative to other terrestrial substrates by mixing of organic matter of a different age [15] , while the marine bulk organic matter CIE is likely augmented compared with other marine substrates by photosynthetic inputs from terrestrial and marine environments [15] , [28] , [29] , [30] . Variability in the degree of these inputs may explain why bulk marine organic matter shows the greatest variability among all substrates (1 σ =±2.2‰). Within purely terrestrial systems, the median CIE recorded in plant lipids (−5.0‰) reflects the full effects of elevated p CO 2 levels on plant isotope fractionation (as shown here and in [26] ); the similar median CIE recorded in fossil tooth enamel (−4.9‰) is not surprising considering that it reflects the δ 13 C value of the plants the herbivore consumes. The very large CIE measured in paleosol carbonate (average=−5.5‰, median=−6.3‰) may reflect a combination of the enhanced fractionation by plants under high p CO 2 , diffusion of increased p CO 2 levels into the soil and increased productivity. Based on measurements of enamel carbonate, Secord et al. [33] attribute 1.5‰ of the CIE measured in soil carbonate to increased rates of carbon turnover, driven by warmer climate. Our results illustrate the need to account for changes in p CO 2 concentration when interpreting changes in the carbon isotope composition of substrates derived at least in part from C 3 land plants, which dominate the terrestrial carbon record. Although our analysis was applied specifically to the PETM, the fundamental p CO 2 effect and equations presented here can be applied similarly to other global CIE events recorded in marine and terrestrial sediments (for example, Aptian–Albian, Early Toarcian, Triassic–Jurassic, Permian–Triassic and many others) in order to quantitatively reconstruct levels of p CO 2 before and during the CIE event. Quantifying Δ p CO 2 We used the following mass balance equation modified from McInerney and Wing [11] to quantify Δ p CO 2 for each of the proposed sources (vertical, coloured lines in Fig. 3 : green=methane hydrate [14] , δ 13 C source =−60‰; purple=thermogenic methane [54] or permafrost thawing [50] , δ 13 C source =−30‰; and orange=wildfire burning [55] or oxidation of organic matter from drying of epicontinental seas [56] , δ 13 C source =−22‰): where M inital is the mass of the Palaeocene surface reservoir, δ 13 C final is the δ 13 C value at the PETM (δ 13 C final =δ 13 C initial +CIE marine ), δ 13 C initial is the δ 13 C value of the Late Palaeocene carbon pool and δ 13 C source is the δ 13 C value of the source responsible for the CIE. We used CIE marine (and not CIE terrestrial ) because it does not incorporate any land-plant-derived components and thus only represents changes in δ 13 C CO2 . The constant 0.3 indicates that for every 1 Pg C added p CO 2 increases 0.3 p.p.m.v. ( [11] ); this value is within the range of values suggested from models of the carbon release at the PETM (for example, 0.23–0.39; [12] , [27] , [57] ). We calculated the value for CIE marine (−2.6‰) as the average of the CIEs measured in benthic forams (−2.5±1.0‰, n =36), planktic forams (−2.7±1.0‰, n =36) and bulk marine carbonate (−2.7±1.1‰, n =33) as listed in Table 1 of McInerney and Wing [11] . Bulk marine organic matter (CIE=−4.1±2.2‰, n =11) was not included in the average because it may contain a mix of marine and terrestrial inputs [28] , [29] , [30] ; the single CIE measured on algal lipids (CIE=−3.5‰) was also excluded. Our values for M initial =50,000 Pg C and δ 13 C initial =−2.5‰ were based on the values used by McInerney and Wing [11] . We note, however, that the value for δ 13 C initial =−2.5‰ may be too low; we estimate δ 13 C initial as high as −0.1‰ assuming a pre-industrial value of −2.1 to −2.6‰ ( [14] ) offset by +2.0‰ based on the secular change in δ 13 C ( [58] ). How to cite this article: Schubert, B. A. & Jahren, A. H. Reconciliation of marine and terrestrial carbon isotope excursions based on changing atmospheric CO 2 levels. Nat. Commun. 4:1653 doi: 10.1038/ncomms2659 (2013).